Pathological α-synuclein impairs adult-born granule cell development and functional integration in the olfactory bulb Although the role of noxious α-synuclein (α-SYN) in the degeneration of midbrain dopaminergic neurons and associated motor deficits of Parkinson’s disease is recognized, its impact on non-motor brain circuits and related symptoms remains elusive. Through combining in vivo two-photon imaging with time-coded labelling of neurons in the olfactory bulb of A30P α-SYN transgenic mice, we show impaired growth and branching of dendrites of adult-born granule cells (GCs), with reduced gain and plasticity of dendritic spines. The spine impairments are especially pronounced during the critical phase of integration of new neurons into existing circuits. Functionally, retarded dendritic expansion translates into reduced electrical capacitance with enhanced intrinsic excitability and responsiveness of GCs to depolarizing inputs, while the spine loss correlates with decreased frequency of AMPA-mediated miniature EPSCs. Changes described here are expected to interfere with the functional integration and survival of new GCs into bulbar networks, contributing towards olfactory deficits and related behavioural impairments. The olfactory bulb (OB) constitutes the first central hub for the processing of odour inputs and represents one of few brain structures constantly supplied with adult-born neurons. Throughout adulthood, this area receives neuronal precursors from the subventricular zone (SVZ) via the rostral migratory stream (RMS), which differentiate into local interneurons and incorporate into existing networks. Despite that the majority of the new arrivals fail to integrate and undergo apoptosis, these cells appear to comprise more than half of the total population of local interneurons in the mature bulb [1] . It emerges that the process of integration of adult-born neurons depends on the activity of local circuits [2] , with extrinsic inputs critically influencing their survival [1] , [3] , [4] . Indeed, the deficit of both sensory and sub-cortical drives is known to disrupt the recruitment of neuronal precursors into functional assemblies [5] . Although mitral and tufted cells (MCs and TCs) hold the central positions in the OB circuitry and are in charge of the primary processing and integration of sensory inputs, the functional dynamics of bulbar networks and the efferent code transmitted to downstream targets are constantly adjusted by the local interneurons [6] , [7] . The unusually high ratio of interneuron—principal cell (100:1) in this forebrain region with their strong reciprocal connections testify the physiological importance of the former, represented largely by dopaminergic and GABAergic periglomerular cells and GABAergic granule cells (GCs) [8] , [9] , [10] . Importantly, latter comprise the vast majority (>90%) of local interneurons and represent the predominant fraction of bulbar adult-born neurons [1] . Positioned in the core of the OB, GCs extend their apical dendrites into the external plexiform layer to form dendro-dendritic synapses with MCs/TCs. Of note, each synapse between a GC spine and lateral dendrite of the principal neuron contains reciprocal specializations for transmitter release [11] , [12] . As a result of such unique arrangement, depolarization of the MC (and TC) dendrite activates the secretion of glutamate onto GC spines, which in turn release GABA back onto these neurons, providing a cellular basis for recurrent and lateral inhibition [13] essential for odour discrimination and evaluation of its adaptive significance. Thus, to become fully engaged into the functional circuitry of the OB, the adult-born GCs face a daunting task—impeccable integration into the existing circuits, to ensure the uninterrupted functioning of the bulbar neuronal assemblies. Over the recent years, significant efforts have been made to identify the sequences of cellular and molecular events underpinning the processes of recruitment, maturation and integration of adult-born neurons in the OB [4] , [14] , [15] . While major progress has been made towards interpreting the basic biology and physiological mechanisms of GCs and their role in processing of olfactory inputs, little is known about the synaptic functions and plasticity of adult-born GCs under pathological conditions. Here, we focus on investigating the impact of aggregation-prone A30P α-synuclein (α-SYN) on the development of new GCs and the functionality of dendro-dendritic synapses, with the aim of identifying the cause for the reduced survival of these neurons in the OB of transgenic α-SYN mice [5] . A detailed analysis of the morphological and functional changes of new GCs may deepen our understanding of the mechanisms of synaptic dysfunction and neurodegeneration in the OB. Reduced survival of adult-born GCs in A30P α-SYN mice Excessive deposition of hyperphosphorylated α-SYN in Lewy bodies in the brain constitutes one of the key histopathological hallmarks of Parkinson’s disease (PD) [16] . In the forebrain, the Lewy Body pathology initiates in the OB and correlates with early-onset olfactory deficit [17] , [18] , [19] . Although adult neurogenesis in the human OB remains a matter of controversy [20] , [21] , [22] , in rodents, ample evidence suggest that olfaction depends on the uninterrupted supply of newborn neurons to the existing networks [1] , [2] , [3] , [4] , [5] , [7] , [8] , [9] . In A30P α-SYN mice, overexpressing aggregation-prone α-SYN under control of the Thy1 promoter [23] , [24] , considerable depositions of this protein were found in OB principal cells and interneurons, with MCs showing the pathology-associated α-SYN phosphorylation [25] . We first examined whether this excess of α-SYN affects the maturation and survival of adult-born GCs in 6-month-old mice ( Fig. 1d–i ). Immunolabelling of newborn cells in the SVZ with bromodeoxyuridine (BrdU) ( Fig. 1a,b ) and subsequent cell counting revealed no differences in the number of BrdU-positive cells in the SVZ of A30P α-SYN (138.000±28.300 cells mm −3 ; n =3) or control mice (148.000±35.000 cells mm −3 ; n =3; P =0.894; Fig. 1c ), implying no alterations in neuronal proliferation. However, double immunofluorescence analysis of OB slices with the neuron-specific nuclear protein NeuN and adult-born neuron marker BrdU revealed ~44.5% less new GCs after 1 month (32 days) in A30P α-SYN mice compared with control (BrdU/NeuN per total NeuN: 2.0±0.1%, n =6 versus 3.6±0.5%, n =5, P =0.0081; Fig. 1d,e ). Interestingly, quantitative analysis of neuron survival after 21 days showed ~21.2% less immature GCs in A30P α-SYN mice compared with control (BrdU/NeuN per total NeuN: 3.3±0.1%, n =5 versus 2.6±0.1%, n =5, P =0.0097; Fig. 1f,g ). Likewise, the number of cells labelled for doublecortin (DCX), a microtubule-associated protein almost exclusively expressed in migrating neuroblasts and immature neurons, was reduced by ~33.3% in A30P α-SYN mice compared with controls (DCX-positive cells mm −3 : 34,000±4,100, n =6 versus 51,000±5,200, n =6, P =0.0263; Fig. 1h,i ). The stronger decrease in the fraction of mature adult-born GCs compared with immature precursors in the GC layer suggests the maturation process as the critical step for the survival of new neurons in A30P α-SYN mice. Similar analysis with comparison of the cell proliferation and survival of adult-born GCs in α-SYN knockout (KO) mice showed that the lack of α-SYN did not alter their proliferation (139,000±16,400 cells mm −3 ; n =3; P =0.919, Fig. 1b,c ) or survival (BrdU/NeuN per total NeuN: 2.7±0.3% BrdU/NeuN, n =6; P =0.148, Fig. 1d,e ). 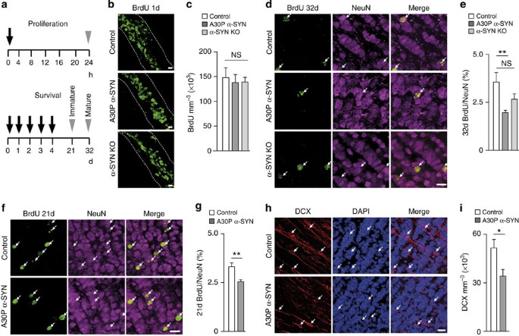Figure 1: Reduced survival of adult-born GCs in A30P α-SYN mice. (a) Schematic of the experimental protocol used for the analysis of proliferation (top) and neuron survival (bottom) in 6-month-old control, A30P α-SYN and α-SYN KO mice. Black arrows indicate time points of BrdU-injection while grey arrowheads show time points of perfusion, followed by immunohistochemistry. (b) Immunofluorescent images of neuronal precursor cells (BrdU, green) in the SVZ in control, A30P α-SYN and α-SYN KO mice: z-stack projections of confocal series. Scale bar, 10 μm. (c) Summary plots of the number of BrdU-labelled cells mm−3SVZ in all three groups (n=3 mice per group;P=0.894 for control/A30P α-SYN;P=0.919 for control/α-SYN KO;P=0.998 for A30P α-SYN/α-SYN KO). (d) Immunofluorescent micrographs of mature, ~32-day-old adult-born (BrdU, green) neurons (NeuN, magenta) in the OB GC layer in control, A30P α-SYN and α-SYN KO mice: z-stack projections of confocal series. White arrows point to soma of double-labelled (adult-born) GCs (merge). Scale bar, 10 μm. (e) Summary plots showing the percentage of BrdU/NeuN-labelled neurons in the GC layer of control, A30P α-SYN and α-SYN KO mice (n=5, 6 and 6 mice per group, respectively;P=0.0081 for control/A30P α-SYN;P=0.148 for control/α-SYN KO;P=0.260 for A30P α-SYN/α-SYN KO). (f) Immunofluorescent images of immature, ~21-day-old adult-born (BrdU, green) neurons (NeuN, magenta) in the GC layer in control and A30P α-SYN mice: z-stack projections of confocal series. White arrows point to soma of double-labelled (adult-born) GCs (merge). Scale bar, 10 μm. (g) Summary plots demonstrating the percentage of BrdU/NeuN-labelled neurons in the GC layer of both groups (n=5 mice per group;P=0.0097). (h) Immunofluorescent images of immature (DCX, red) adult-born GCs in sections counterstained with DAPI (blue) in control and A30P α-SYN mice: z-stack projections of confocal series. White arrows point to cell bodies of some immature GCs. Scale bar, 10 μm. (i) Summary plots of the numbers of DCX-positive GCs mm−3in both groups (n=6 mice per group;P=0.0263). Values are presented as mean±s.e.m. One-way analysis of variance/Tukey–Kramerpost hoctest (c,e); Student’st-test (g,i). Figure 1: Reduced survival of adult-born GCs in A30P α-SYN mice. ( a ) Schematic of the experimental protocol used for the analysis of proliferation (top) and neuron survival (bottom) in 6-month-old control, A30P α-SYN and α-SYN KO mice. Black arrows indicate time points of BrdU-injection while grey arrowheads show time points of perfusion, followed by immunohistochemistry. ( b ) Immunofluorescent images of neuronal precursor cells (BrdU, green) in the SVZ in control, A30P α-SYN and α-SYN KO mice: z-stack projections of confocal series. Scale bar, 10 μm. ( c ) Summary plots of the number of BrdU-labelled cells mm −3 SVZ in all three groups ( n =3 mice per group; P =0.894 for control/A30P α-SYN; P =0.919 for control/α-SYN KO; P =0.998 for A30P α-SYN/α-SYN KO). ( d ) Immunofluorescent micrographs of mature, ~32-day-old adult-born (BrdU, green) neurons (NeuN, magenta) in the OB GC layer in control, A30P α-SYN and α-SYN KO mice: z-stack projections of confocal series. White arrows point to soma of double-labelled (adult-born) GCs (merge). Scale bar, 10 μm. ( e ) Summary plots showing the percentage of BrdU/NeuN-labelled neurons in the GC layer of control, A30P α-SYN and α-SYN KO mice ( n =5, 6 and 6 mice per group, respectively; P =0.0081 for control/A30P α-SYN; P =0.148 for control/α-SYN KO; P =0.260 for A30P α-SYN/α-SYN KO). ( f ) Immunofluorescent images of immature, ~21-day-old adult-born (BrdU, green) neurons (NeuN, magenta) in the GC layer in control and A30P α-SYN mice: z-stack projections of confocal series. White arrows point to soma of double-labelled (adult-born) GCs (merge). Scale bar, 10 μm. ( g ) Summary plots demonstrating the percentage of BrdU/NeuN-labelled neurons in the GC layer of both groups ( n =5 mice per group; P =0.0097). ( h ) Immunofluorescent images of immature (DCX, red) adult-born GCs in sections counterstained with DAPI (blue) in control and A30P α-SYN mice: z-stack projections of confocal series. White arrows point to cell bodies of some immature GCs. Scale bar, 10 μm. ( i ) Summary plots of the numbers of DCX-positive GCs mm −3 in both groups ( n =6 mice per group; P =0.0263). Values are presented as mean±s.e.m. One-way analysis of variance/Tukey–Kramer post hoc test ( c , e ); Student’s t -test ( g , i ). Full size image Sparse branching of apical GC dendrites in A30P α-SYN mice The dynamics of the development of adult-born GC dendrites with high levels of structural plasticity in normal mouse brains are well described [26] . To gain insights as to whether the excessive load of aggregation-prone A30P α-SYN in the OB neurons affects the development of adult-born GCs, we estimated the total length and branching of apical and basal dendrites as well as the somata size by genetic pre-labelling of GCs, using established methodology [27] . Four weeks after injection of enhanced green fluorescent protein (eGFP)-encoding lentivirus (LV) into the RMS, 6-month-old mice were perfused and eGFP-labelled GCs were fully reconstructed from confocal image stacks with Neurolucida ( Fig. 2a ). While there was a tendency for reduced total dendritic lengths in A30P α-SYN mice as compared with controls (691±78 μm; n =7 versus 804±50 μm; n =6 mice), the inter-group differences failed to reach statistical significance ( P =0.241; Fig. 2b ). Interestingly, however, the length of distal apical dendrites was significantly reduced in A30P α-SYN mice (381±59 μm; n =7 mice) compared with controls (538±29 μm; n =6 mice; P =0.0206; Fig. 2c ). Analysis of the dendritic branching per individual tree of adult-born GCs demonstrates that this parameter was reduced in A30P α-SYN mice compared with controls (4.5±0.6; n =7 versus 6.5±0.6; n =6 mice, P =0.0296; Fig. 2d ). Similar measurements pulled from α-SYN KO mice showed neither total dendritic length (737±36 μm; n =5 mice, P =0.637) and apical dendritic length (441±29 μm; n =5 mice; P =0.304) nor their branching points (6.9±1.0; n =5 mice, P =0.186) being significantly altered ( Fig. 2a–d ). Soma perimeter analysis also showed comparable values for all three groups ( Fig. 2e ; P =0.981 for control/A30P α-SYN; P =0.990 for control/α-SYN KO; P =0.999 for A30P α-SYN/α-SYN KO). 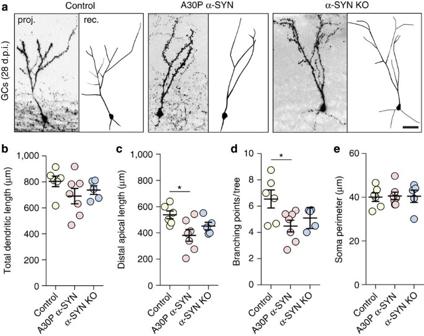Figure 2: Reduced expansion and branching of adult-born GC apical dendrites in A30P α-SYN mice. (a) Representative micrographs of adult-born GCs LV transduced with eGFP at 28 days post injection (d.p.i.): confocal z-stack projections (left) with their complete reconstruction (right) in control, A30P α-SYN and α-SYN KO mice. Scale, 20 μm. Note considerably reduced branching of apical dendrites in A30P α-SYN mice. (b–e) Summary graphs quantifying the size of adult-born GCs in control, A30P α-SYN and α-SYN KO mice (n=6, 7 and 5 mice per group, respectively), with (b) total dendritic length (P=0.241 for control/A30P α-SYN;P=0.637 for control/α-SYN KO;P=0.792 for A30P α-SYN/α-SYN KO), (c) distal apical dendritic length (P=0.0206 for control/A30P α-SYN;P=0.304 for control/α-SYN KO;P=0.407 for A30P α-SYN/α-SYN KO), (d) number of branching points per apical dendritic tree (P=0.0296 for control/A30P α-SYN;P=0.186 for control/α-SYN KO;P=0.703 for A30P α-SYN/α-SYN KO) and (e) soma perimeter (P=0.981 for control/A30P α-SYN;P=0.990 for control/α-SYN KO;P=0.999 for A30P α-SYN/α-SYN KO). Values are presented as mean±s.e.m. One-way analysis of variance/Tukey–Kramerpost hoctest. Figure 2: Reduced expansion and branching of adult-born GC apical dendrites in A30P α-SYN mice. ( a ) Representative micrographs of adult-born GCs LV transduced with eGFP at 28 days post injection (d.p.i. ): confocal z-stack projections (left) with their complete reconstruction (right) in control, A30P α-SYN and α-SYN KO mice. Scale, 20 μm. Note considerably reduced branching of apical dendrites in A30P α-SYN mice. ( b – e ) Summary graphs quantifying the size of adult-born GCs in control, A30P α-SYN and α-SYN KO mice ( n =6, 7 and 5 mice per group, respectively), with ( b ) total dendritic length ( P =0.241 for control/A30P α-SYN; P =0.637 for control/α-SYN KO; P =0.792 for A30P α-SYN/α-SYN KO), ( c ) distal apical dendritic length ( P =0.0206 for control/A30P α-SYN; P =0.304 for control/α-SYN KO; P =0.407 for A30P α-SYN/α-SYN KO), ( d ) number of branching points per apical dendritic tree ( P =0.0296 for control/A30P α-SYN; P =0.186 for control/α-SYN KO; P =0.703 for A30P α-SYN/α-SYN KO) and ( e ) soma perimeter ( P =0.981 for control/A30P α-SYN; P =0.990 for control/α-SYN KO; P =0.999 for A30P α-SYN/α-SYN KO). Values are presented as mean±s.e.m. One-way analysis of variance/Tukey–Kramer post hoc test. Full size image Impaired development of dendritic spines in adult-born GCs Next, we turned on the assessment of the spine density in adult-born GCs ( Fig. 3 ). As the density of apical dendritic spines in these neurons provides direct anatomical readout for dendro-dendritc synapses [28] , any difference between this parameter in A30P α-SYN mice and controls would imply changes of the development and structural plasticity, with potential implication for olfactory functions. Consistent with reports from other brain regions [29] , in younger (3-month-old) control mice the spine density of OB GCs (28 days post injection) was higher than in age-matched GCs in older (6-month-old) animals (0.81±0.02 spines μm −1 ; n =6 versus 0.66±0.09 spines μm −1 ; n =6 mice; P =0.0174; Fig. 3a,b ). Similar assessments of the spine density in adult-born GCs in 3-month-old A30P α-SYN mice revealed ~7.4% reduction (0.75±0.02 spines μm −1 ; n =5 mice) compared with age-matched controls ( P =0.0100; Fig. 3b ). These changes became stronger at 6 months of age, with A30P α-SYN mice showing ~22.8% decrease in spine density (0.51±0.04 spines μm −1 dendrite; n =6 mice) compared with controls (0.66±0.09 spines μm −1 ; n =6 mice; P =0.0187; Fig. 3a,b ). It is worth stressing that the density of apical dendritic spines in age-matched α-SYN KO mice (0.62±0.11 spines μm −1 ; n =6) did not differ from controls ( P =0.752) or A30P α-SYN mice ( P =0.0751; Fig. 3b ). To establish whether the decline in spine density in 6-month-old A30P α-SYN mice is a persistent trait, we analysed the apical spines of adult-born GCs at two additional neuro-developmental stages (2 and 8 weeks) ( Fig. 3c,d ). Interestingly, no difference was found between 2-week-old GCs of A30P α-SYN and control mice (0.48±0.04 spines μm −1 ; n =3 versus 0.44±0.04 spines μm −1 ; n =4; P =0.272), with the spine density being the lowest at this early developmental stage ( Fig. 3d ). Differently, at 8 weeks, the density of spines in controls exceeded that of A30P α-SYN mice (0.60±0.03 spines μm −1 ; n =3 versus 0.53±0.04 spines μm −1 ; n =5, P =0.0459; Fig. 3c ). Overall, these findings suggest a considerable reduction of dendritic spines during the critical window of development and integration [30] , [31] of adult-born GCs in A30P α-SYN mice. 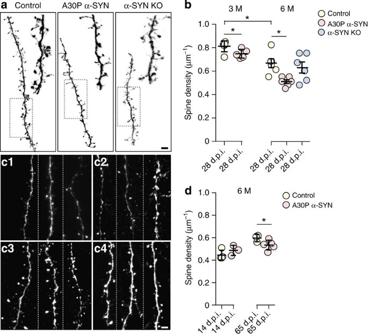Figure 3: Lowered dendritic spine density in adult-born GCs of A30P α-SYN mice. (a) Representative high-resolution micrographs of the apical dendritic segments of adult-born GCs LV transduced with eGFP at 28 days post injection (d.p.i.): confocal z-stack projections. Six-month-old control, age-matched A30P α-SYN and α-SYN KO mice. Scale bar, 5 μm. (b) Summary graphs quantifying the dendritic spine density of adult-born GCs (28 d.p.i.) in 3-month-old control and A30P α-SYN mice (n=6 and 5 mice per group, respectively; left panel;P=0.0100) and 6-month-old control, A30P α-SYN and α-SYN KO mice (n=6 mice per group; right panel;P=0.0187 for control/A30P α-SYN;P=0.752 for control/α-SYN KO;P=0.0751 for A30P α-SYN/α-SYN KO). Please note the stronger reduction in the spine density of the older A30P α-SYN mice when compared with controls. (c) Representative micrographs of the apical dendritic segments of adult-born GCs LV transduced with eGFP at 14 d.p.i. in control (c1), A30P α-SYN mice (c2) and at 65 d.p.i. in control (c3) and A30P α-SYN mice (c4): confocal z-stack projections. Mice were 6 months old. Scale bar, 5 μm. (d) Similar measurements from adult-born GCs at 14 and 65 d.p.i. in 6-month-old control and A30P α-SYN mice (n=3 and 4 mice per group;P=0.272 at 14 d.p.i.;P=0.0459 at 65 d.p.i.). Values are presented as mean±s.d. One-way analysis of variance/Tukey–Kramerpost hoctest (b); Student’st-test (b,d). Figure 3: Lowered dendritic spine density in adult-born GCs of A30P α-SYN mice. ( a ) Representative high-resolution micrographs of the apical dendritic segments of adult-born GCs LV transduced with eGFP at 28 days post injection (d.p.i. ): confocal z-stack projections. Six-month-old control, age-matched A30P α-SYN and α-SYN KO mice. Scale bar, 5 μm. ( b ) Summary graphs quantifying the dendritic spine density of adult-born GCs (28 d.p.i.) in 3-month-old control and A30P α-SYN mice ( n =6 and 5 mice per group, respectively; left panel; P =0.0100) and 6-month-old control, A30P α-SYN and α-SYN KO mice ( n =6 mice per group; right panel; P =0.0187 for control/A30P α-SYN; P =0.752 for control/α-SYN KO; P =0.0751 for A30P α-SYN/α-SYN KO). Please note the stronger reduction in the spine density of the older A30P α-SYN mice when compared with controls. ( c ) Representative micrographs of the apical dendritic segments of adult-born GCs LV transduced with eGFP at 14 d.p.i. in control ( c1 ), A30P α-SYN mice ( c2 ) and at 65 d.p.i. in control ( c3 ) and A30P α-SYN mice ( c4 ): confocal z-stack projections. Mice were 6 months old. Scale bar, 5 μm. ( d ) Similar measurements from adult-born GCs at 14 and 65 d.p.i. in 6-month-old control and A30P α-SYN mice ( n =3 and 4 mice per group; P =0.272 at 14 d.p.i. ; P =0.0459 at 65 d.p.i.). Values are presented as mean±s.d. One-way analysis of variance/Tukey–Kramer post hoc test ( b ); Student’s t -test ( b , d ). Full size image Reduced GC spine density and stability in vivo To obtain a more comprehensive picture of the spine dynamics during maturation, apical dendrites of eGFP-labelled GCs were imaged over several days in vivo using two-photon microscopy ( Fig. 4a–c ). In two independent cohorts of 6-month-old mice, spine density and turnover were analysed with numbers of gained, stable and lost spines quantified at early (21–25 days post injection; d.p.i.) and late (28–44 d.p.i.) maturation stages. To avoid possible variance in the age of labelled adult-born GCs caused by transfection of faster and slower dividing precursors, viral vectors were exclusively injected into the RMS [26] , [27] . Progressive increase in the spine density was revealed in controls (0.54±0.05 spines μm −1 versus 0.65±0.07 spines μm −1 , 21 and 25 d.p.i., respectively, n =5; P =0.0084), an observation that contrasts with the relatively invariable density of spines in GCs of A30P α-SYN mice over the same period of time (0.47±0.07 spines μm −1 versus 0.45±0.08 spines μm −1 , n =3; P =0.650; Fig. 4d ). This discrepancy is readily reflected in deviation of the mean values of spine densities, with the difference becoming statistically significant from 23 d.p.i. ( P =0.0054) and persisting over the two following time points ( P =0.0090 at 24 d.p.i., P =0.0007 at 25 d.p.i. ; Fig. 4d ). Similar trend has become evident from fractional comparison of the spine densities over later time points with the initial, with both, increase in spine density ( P =0.0116) and inter-genotype differences ( P =0.0143) becoming larger with age ( Fig. 4e ). Remarkably, assessment of the spine turnover rate between 21 and 25 d.p.i. showed this parameter being relatively stable in both genotypes ( P =0.999; Fig. 4f ), while the spine stability analysis highlighted its decrease in A30P α-SYN mice compared with controls (0.40±0.05 spines μm −1 versus 0.32±0.04 spines μm −1 at 24 d.p.i. and 0.46±0.04 spines μm −1 versus 0.28±0.03 spines μm −1 at 25 d.p.i. ; P =0.0499 and P =0.0001; Fig. 4g ). This observation was corroborated by comparison of the survival rate of dendritic spines in the two genotypes ( Fig. 4h ). Indeed, while 58.1±3.0% spines counted in controls at 21 d.p.i. were still preserved at 25 d.p.i., this number was reduced to 44.0±1.5% in the A30P α-SYN mice ( P =0.0002). Similar experiments with analysis of the spine dynamics in the second cohort of mice between 28 and 44 d.p.i. revealed no further changes in the spine density in both control and A30P α-SYN mice (at 44 d.p.i. ; 0.51±0.07 spines μm −1 , n =4 versus 0.37±0.04 spines μm −1 ; n =5, respectively; P =0.276; Fig. 4d,e ), with gradual decrease in spine turnover being recorded in both genotypes ( P =0.0410; Fig. 4f ). Taken as a whole, our in vivo imaging data suggest impairment of the gain and stability of dendritic spines during adult-born GC maturation in A30P α-SYN mice. 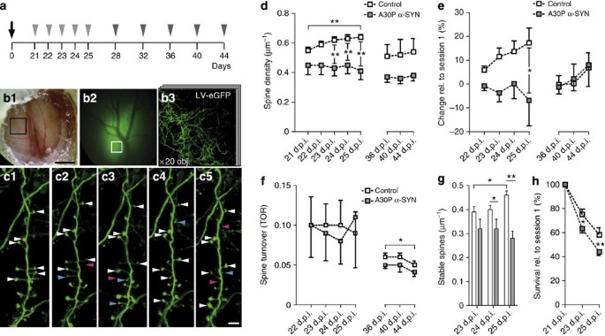Figure 4:Impaired dendritic spine density and stabilization in adult-born GCs of A30P α-SYN micein vivo. (a) A schematic of the experimental protocol indicating the time points of LV injection with OB craniotomy (black arrow) followed byin vivotwo-photon imaging in two cohorts of mice (light and dark grey arrowheads). (b1–3) Experimental setup for chronic two-photon imaging of eGFP-expressing adult-born GCs through open-skull cranial windows implanted over both OBs. (b1) A dorsal view of the craniotomy with a black box defining the region of interest presented in (b2) with distinct shadows of reference blood vessels visible. Scale bar, 1 mm (b1). (b3) Low-magnification two-photon micrograph of the region of interest with eGFP-labelled live dendrites. (c1–5) Time-lapse series of a typical dendritic segment of the adult-born GC in the external plexiform layer (21–25 d.p.i.). Arrowheads point to stable (white), gained (blue) and lost (magenta) spines. Scale bar, 5 μm. (d) Quantification of the dendritic spine density in adult-born GCs at various time points in control and A30P α-SYN mice (first cohort:n=8;P=0.0054 at 23 d.p.i.;P=0.0090 at 24 d.p.i.;P=0.0007 at 25 d.p.i., with increase in controlP=0.0084; second cohort:n=9;P=0.412 at 36 d.p.i.;P=0.276 at 40 and 44 d.p.i.). (e) A summary graph illustrating fractional changes in the spine density relative to the first imaging session in both genotypes (first cohort:n=8;P=0.0143 at 25 d.p.i., second cohort:n=9;P=0.999 at 44 d.p.i.). (f–h) Graphical representation of the (f) dendritic spine turnover (first cohort:n=8;P=0.999; second cohort:n=9;P=0.743, with gradual decrease in both groupsP=0.0410), (g) stabilization (first cohort:n=8;P=0.0499 at 24 d.p.i. andP=0.001 at 25 d.p.i., with increase in controlP=0.0471) and (h) survival (first cohort:n=8;P=0.015 at 23 d.p.i. andP=0.0002 at 25 d.p.i.). Note that the fraction of survived spines is expressed relative to the first imaging session taken as 100%. Values are presented as mean±s.e.m. One-way analysis of variance (ANOVA)/Tukey–Kramerpost hoctest (d,f,g); two-way ANOVA/Bonferronipost hoctest (d,e,g,h). Figure 4: Impaired dendritic spine density and stabilization in adult-born GCs of A30P α-SYN mice in vivo . ( a ) A schematic of the experimental protocol indicating the time points of LV injection with OB craniotomy (black arrow) followed by in vivo two-photon imaging in two cohorts of mice (light and dark grey arrowheads). ( b1 – 3 ) Experimental setup for chronic two-photon imaging of eGFP-expressing adult-born GCs through open-skull cranial windows implanted over both OBs. ( b1 ) A dorsal view of the craniotomy with a black box defining the region of interest presented in ( b2 ) with distinct shadows of reference blood vessels visible. Scale bar, 1 mm ( b1 ). ( b3 ) Low-magnification two-photon micrograph of the region of interest with eGFP-labelled live dendrites. ( c1 – 5 ) Time-lapse series of a typical dendritic segment of the adult-born GC in the external plexiform layer (21–25 d.p.i.). Arrowheads point to stable (white), gained (blue) and lost (magenta) spines. Scale bar, 5 μm. ( d ) Quantification of the dendritic spine density in adult-born GCs at various time points in control and A30P α-SYN mice (first cohort: n =8; P =0.0054 at 23 d.p.i. ; P =0.0090 at 24 d.p.i. ; P =0.0007 at 25 d.p.i., with increase in control P =0.0084; second cohort: n =9; P =0.412 at 36 d.p.i. ; P =0.276 at 40 and 44 d.p.i.). ( e ) A summary graph illustrating fractional changes in the spine density relative to the first imaging session in both genotypes (first cohort: n =8; P =0.0143 at 25 d.p.i., second cohort: n =9; P =0.999 at 44 d.p.i.). ( f – h ) Graphical representation of the ( f ) dendritic spine turnover (first cohort: n =8; P =0.999; second cohort: n =9; P =0.743, with gradual decrease in both groups P =0.0410), ( g ) stabilization (first cohort: n =8; P =0.0499 at 24 d.p.i. and P =0.001 at 25 d.p.i., with increase in control P =0.0471) and ( h ) survival (first cohort: n =8; P =0.015 at 23 d.p.i. and P =0.0002 at 25 d.p.i.). Note that the fraction of survived spines is expressed relative to the first imaging session taken as 100%. Values are presented as mean±s.e.m. One-way analysis of variance (ANOVA)/Tukey–Kramer post hoc test ( d , f , g ); two-way ANOVA/Bonferroni post hoc test ( d , e , g , h ). Full size image Selective loss of GABAergic component in apical GC dendrites The head of the spine with GABAergic effector and glutamatergic receptor elements provides the sole output of GCs [12] , [32] . As a bilateral synapse, this structure accommodates exocytotic machinery for the release of GABA and receptive components for sensing glutamate discharged from the lateral dendrites of MCs/TCs. To establish how developmental alterations of dendritic spines of adult-born GCs in A30P α-SYN mice impact the synaptic machinery at this junction, we analysed the levels of vesicular GABA transporter (VGAT) (presynaptic) and gephyrin (postsynaptic) GABAergic synaptic markers in A30P α-SYN mice and compared with controls ( Fig. 5 ). As illustrated, the number of VGAT-positive clusters co-localized with eGFP-labelled spines along individual apical dendrites in A30P α-SYN mice was considerably reduced (1.5±0.1 μm −1 , n =6, versus 2.2±0.3 μm −1 , n =5; P =0.0270; Fig. 5a,b ). Analogous assessments of the level of gephyrin revealed equal distribution of this postsynaptic qualifier protein between the two genotypes (0.7±0.1 μm −1 , n =4 versus 0.9±0.1 μm −1 , n =6; control and A30P α-SYN, respectively; P =0.244), suggesting selective impairment of presynaptic elements of dendro-dendritic GABAergic synapses ( Fig. 5c,d ). This rather unexpected finding prompted us to examine the expression of α-amino-3-hydroxy-5-methyl-4-isoxazolepropionic acid (AMPA) glutamate receptor by quantifying the GluR1-labelled receptor clusters co-localized with eGFP-positive dendrites ( Fig. 5e,f ). These data also provide further insight into state and integrity of dendro-dendritic connections between adult-born GCs and MCs/TCs in A30P α-SYN mice. Similar to gephyrin, expression of GluR1 clusters on dendrites were indistinguishable between the two genotypes (0.19±0.04 μm −1 , n =5 versus 0.20±0.03 μm −1 , n =5, control and A30P α-SYN, respectively; P =0.559). In light of the reduced dendritic spine density on adult-born GCs in A30P α-SYN mice, these findings suggest increased occurrence of AMPA-receptor clusters in remaining reciprocal synapses. It is interesting to note that the analysis of the dendritic spine morphology ( Supplementary Fig. 1c ) revealed a trend towards an increase in the width of the spine head in A30P α-SYN (0.52±0.02; n =14 dendrites) compared with control (0.46±0.01; n =18 dendrites; P =0.08). 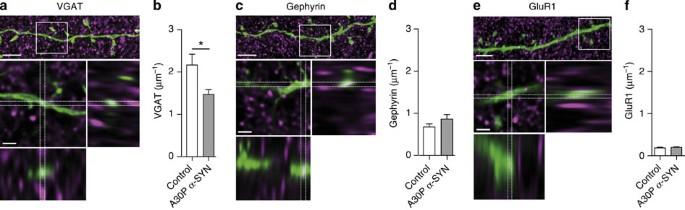Figure 5: Loss of presynaptic GABAergic component on GC apical dendrites in A30P α-SYN mice. (a,c,e) Representative confocal z-stack projections of apical dendritic segment of LV-transduced adult-born GCs (28 days post injection, green) counterstained for (a) VGAT, (c) gephyrin and (e) GluR1 subunit of the AMPA receptor colour code refers toa,cande. Scale bar, 5 μm. Side views illustrate co-localization spots (white) of co-labelled proteins of interest with an eGFP-positive dendritic segment: enlarged from the defined above region (white rectangle). Scale bar, 1.5 μm. Summary plots demonstrating the number of (b) VGAT, (d) gephyrin and (f) GluR1 co-localization spots (μm−1); GC dendrite in control and A30P α-SYN mice (n=5 mice per group;P=0.0270 in (b);P=0.244 in (d);P=0.559 in (f). Values are presented as mean±s.e.m. Student’st-test. Figure 5: Loss of presynaptic GABAergic component on GC apical dendrites in A30P α-SYN mice. ( a , c , e ) Representative confocal z-stack projections of apical dendritic segment of LV-transduced adult-born GCs (28 days post injection, green) counterstained for ( a ) VGAT, ( c ) gephyrin and ( e ) GluR1 subunit of the AMPA receptor colour code refers to a , c and e . Scale bar, 5 μm. Side views illustrate co-localization spots (white) of co-labelled proteins of interest with an eGFP-positive dendritic segment: enlarged from the defined above region (white rectangle). Scale bar, 1.5 μm. Summary plots demonstrating the number of ( b ) VGAT, ( d ) gephyrin and ( f ) GluR1 co-localization spots (μm −1 ); GC dendrite in control and A30P α-SYN mice ( n =5 mice per group; P =0.0270 in ( b ); P =0.244 in ( d ); P =0.559 in ( f ). Values are presented as mean±s.e.m. Student’s t -test. Full size image Enhanced intrinsic responsiveness of adult-born GCs To establish the functional impact of A30P α-SYN on adult-born GCs, electrophysiological measurements were undertaken from eGFP-labelled neurons of the GC layer in acute slices ( Fig. 6a ). Passive properties of the GC membrane were examined under the pharmacological blockade of ionotropic glutamatergic and GABAergic input with kynurinate and picrotoxin, respectively, while action potential firing induced by depolarizing currents were monitored before and after pharmacological interventions. Whole-cell recordings showed that with no bias current injection, the majority of eGFP-positive GCs were electrically silent (8/8 control and 10/12 A30P α-SYN; five animals in each group), but could be driven into continuous firing mode by small steady depolarizing currents ( Fig. 6b ). Neither the resting potential (−64.2±3.6 versus −59.4±2.8 mV; P =0.30) nor the amplitude of threshold current required for inducing firing activity (11.1±2 versus 10.0±1.5 pA; P =0.65) differed between the two genotypes ( n =8 and n =10, control and A30P α-SYN). After blockade of both excitatory and inhibitory inputs, the threshold firing rate (4.3±0.6 versus 4.5±0.7 Hz; P =0.83) and the inter-spike interval variability (CV=0.15±0.03 versus CV=0.13±0.06; P =0.71) were comparable between both genotypes. Interestingly, when the excitatory inputs were spared, the variability of the inter-spike interval in A30P α-SYN GCs was larger compared with control GCs (CV=0.31±0.06 versus CV=0.43±0.05; P =0.030 and P =0.0012, respectively). To establish whether this difference could be attributed to a greater impact of excitatory synaptic inputs on the intrinsic voltage dynamics of adult-born GCs, we first compared their active responsiveness from similar hyperpolarized potentials (between −64 and −66 mV). As illustrated ( Fig. 6b,f ), A30P α-SYN neurons fired spikes more readily than control neurons, with threshold current being lower (18.3±1.6 versus 25.0±1.8 pA; P =0.015). The similar voltage threshold for generation of action potentials (−37.6±0.7 versus −38.2±0.5 mV; P =0.48) and spike amplitudes (67.9±2.4 versus 69.1±2.7 mV; P =0.75) in two groups suggests altered passive properties as the possible cause for increased responsiveness of GCs in A30P α-SYN. This was confirmed by measurements of the membrane capacitance and input resistance of control and A30P α-SYN neurons ( n =16 and n =14, respectively; Fig. 6b–e ). As illustrated, the membrane resistance of GCs in A30P α-SYN was higher (1.90±0.13 versus 1.47±0.15 GΩ; P =0.038) while their capacitance was notably reduced (10.2±0.5 versus 12.6±1.0 pF; P =0.034). Taken together, these findings are in agreement of adult-born GCs being electrically more compact, apparently owing to their underdeveloped dendrites. 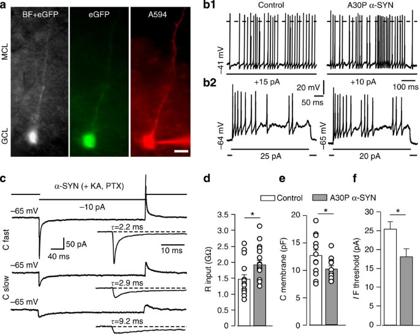Figure 6: Enhanced responsiveness of adult-born GCs in A30P α-SYN mice. (a) Representative micrograph of adult-born GC in acute OB slice: overlie of eGFP and bright field image (left) of eGFP-positive GC before and after loading with A594 (middle and right, respectively) through the patch pipette (bottom-right corner). Scale bar, 10 μm. MLC and GCL—mitral cell layer and granule cell layer, respectively. (b1) Sustained firing activity of adult-born GCs induced by steady supra-threshold depolarizing current: recordings were made in the presence of picrotoxin. Episode of paroxysmal firing were more characteristic to adult-born GCs of A30P α-SYN mice. (b2) Representative evoked spiking of adult-born GCs from hyperpolarized potential (close to −65 mV) demonstrating elevated responsiveness of GCs of A30P α-SYN mice to direct depolarizing stimuli. Note larger injected current and lower number of action potentials in the control (left). (c–e) Assessment of the passive properties of adult-born GCs: (c) capacitative transient recorded in control GC. Currents activated by −5 mV hyperpolarizing voltage pulse from a holding potential of −65 mV: average of five consecutive sweeps. Uncompensated and remaining current after cancellation of the pipette capacitance (top and middle). Bottom—capacitative current after cancellation of the cell capacitance and series resistance compensation (~80%). (d–f) Summary histograms of the input resistance (Rin), membrane capacitance (Cm) and current threshold for inducing action firing from hyperpolarized holding potential in GCs of two genotypes (n=16 and 14 neurons from 5 mice; control and A30P α-SYN, respectively;P=0.038 ind;P=0.033 ine;P=0.015 inf. Open circles indicate the readouts from individual neurons. Values are presented as mean±s.e.m. Student’st-test. Figure 6: Enhanced responsiveness of adult-born GCs in A30P α-SYN mice. ( a ) Representative micrograph of adult-born GC in acute OB slice: overlie of eGFP and bright field image (left) of eGFP-positive GC before and after loading with A594 (middle and right, respectively) through the patch pipette (bottom-right corner). Scale bar, 10 μm. MLC and GCL—mitral cell layer and granule cell layer, respectively. ( b1 ) Sustained firing activity of adult-born GCs induced by steady supra-threshold depolarizing current: recordings were made in the presence of picrotoxin. Episode of paroxysmal firing were more characteristic to adult-born GCs of A30P α-SYN mice. ( b2 ) Representative evoked spiking of adult-born GCs from hyperpolarized potential (close to −65 mV) demonstrating elevated responsiveness of GCs of A30P α-SYN mice to direct depolarizing stimuli. Note larger injected current and lower number of action potentials in the control (left). ( c – e ) Assessment of the passive properties of adult-born GCs: ( c ) capacitative transient recorded in control GC. Currents activated by −5 mV hyperpolarizing voltage pulse from a holding potential of −65 mV: average of five consecutive sweeps. Uncompensated and remaining current after cancellation of the pipette capacitance (top and middle). Bottom—capacitative current after cancellation of the cell capacitance and series resistance compensation (~80%). ( d – f ) Summary histograms of the input resistance ( R in ), membrane capacitance ( C m ) and current threshold for inducing action firing from hyperpolarized holding potential in GCs of two genotypes ( n =16 and 14 neurons from 5 mice; control and A30P α-SYN, respectively; P =0.038 in d ; P =0.033 in e ; P =0.015 in f . Open circles indicate the readouts from individual neurons. Values are presented as mean±s.e.m. Student’s t -test. Full size image Reduced excitatory synaptic inputs substantiate GC spine loss To identify the functional consequences of impaired spine plasticity caused by A30P α-SYN on excitatory synaptic transmission in new GCs in the OB, we measured their sEPSC under the blockade of fast inhibitory synaptic transmission with picrotoxin ( Fig. 7 ). Although the transfer of charge activated by AMPA receptors is the main mechanism underlying the spontaneous fast glutamatergic inputs in neurons, substantial contribution of N -methyl- D -aspartate (NMDA) receptor-dependent currents has also been documented [33] . Comparison of sEPSCs from control and A30P α-SYN GCs revealed no differences between their frequency (8.0±1.2 Hz, n =8 versus 5.9±0.9 Hz, n =12; P =0.21) or amplitude (23.2±3.1 versus 22.7±3.6 pA; P =0.94), although a trend towards lower frequencies was evident in neurons from transgenic mice ( Fig. 7a–c ). This result was surprising in light of the significant reduction in spine density in adult-born GCs. Similar analysis of sEPSCs after the blockade of NMDA receptor-mediated currents with a selective antagonist D-AP5 revealed no considerable change in sEPSC frequency (7.0±1.3 Hz and 5.7±1.3 Hz; control and A30P α-SYN, respectively; P =0.506). Interestingly, such blockade caused a notable decrease in the amplitude of sEPSC currents in adult-born GCs of controls but not A30P α-SYN mice (18.4±1.2 versus 22.7±1.2 pA; P =0.026). Comparison of the kinetic parameters of AMPA-mediated miniature EPSCs (mEPSCs) between two genotypes revealed similar rise and decay time constants ( Supplementary Fig. 2 ). Of note, the estimated values for the vast majority of mEPSCs in both controls and A30P α-SYN mice were close to half of those reported for stimulation-induced slow, presumably dendro-dendritic EPSCs in younger rats [34] , with rare faster events also occasionally detected. Differences between the frequency and amplitude of the two genotypes were revealed on comparison of the mEPSCs after blockade of action potential-dependent synaptic currents by tetrodotoxin (TTX), a selective blocker of Na + channels. In agreement with our morphometric data, adult-born GCs of A30P α-SYN mice displayed considerably reduced mEPSCs frequency (3.7±0.4 Hz, n =8 versus 1.3±0.2 Hz, n =10 neurons; P =0.0001) while their amplitude was significantly enhanced (12.2±0.9 versus 9.2±1.0 pA, respectively; P =0.045; Fig. 7d,e ). Thus, it appears that decrease in the frequency of AMPA-receptor-mediated mEPCSs, possibly due to reduced density of dendritic spines in adult-born GCs, is accompanied with notable increase of their amplitude. 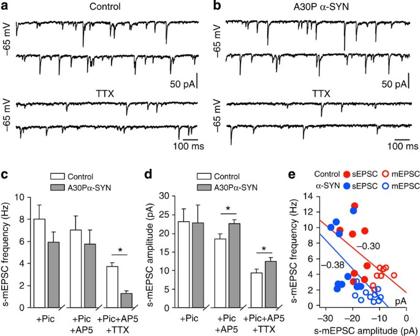Figure 7:Reducedfrequency but larger amplitude of miniature excitatory postsynaptic currents in adult-born GCs of A30P α-SYN mice. (a,b) Comparison of the voltage clamp recordings of sEPSCs (total, upper traces) and mEPSCs (TTX-resistant, lower traces) from adult-born GCs of control and A30P α-SYN mice. (c,d) Summary histograms of spontaneous and miniature (s-m) EPSC frequency (c) and amplitude (d) under the blockade of inhibitory inputs with picrotoxin followed by blockade of the NMDA receptor with D-AP5 and further inhibition of the action potential-dependent fraction of sEPSCs with TTX in both groups (n=8 and 10 neurons from five mice; control and A30P α-SYN, respectively;P=0.210, 0.510 and 0.0001 inc;P=0.920, 0.026 and 0.045 ind; from left to right). Note lower frequency and higher amplitude of TTX-resistant fraction of EPSCs (sEPSCs) in adult-born GCs of A30P α-SYN mice. (e) Graphical representation of the relationship of the AMPA-receptor-mediated sEPSCs and mEPSCs in individual GCs of the two genotypes. Steeper slope of amplitude and frequency relation between sEPSCs and mEPSCs in GCs of A30P α-SYN mice indicates lower sensitivity of the sEPSCs amplitude to TTX. Values are presented as mean±s.e.m. Student’st-test (c,d). Figure 7: Reduced frequency but larger amplitude of miniature excitatory postsynaptic currents in adult-born GCs of A30P α-SYN mice. ( a , b ) Comparison of the voltage clamp recordings of sEPSCs (total, upper traces) and mEPSCs (TTX-resistant, lower traces) from adult-born GCs of control and A30P α-SYN mice. ( c , d ) Summary histograms of spontaneous and miniature (s-m) EPSC frequency ( c ) and amplitude ( d ) under the blockade of inhibitory inputs with picrotoxin followed by blockade of the NMDA receptor with D-AP5 and further inhibition of the action potential-dependent fraction of sEPSCs with TTX in both groups ( n =8 and 10 neurons from five mice; control and A30P α-SYN, respectively; P =0.210, 0.510 and 0.0001 in c ; P =0.920, 0.026 and 0.045 in d ; from left to right). Note lower frequency and higher amplitude of TTX-resistant fraction of EPSCs (sEPSCs) in adult-born GCs of A30P α-SYN mice. ( e ) Graphical representation of the relationship of the AMPA-receptor-mediated sEPSCs and mEPSCs in individual GCs of the two genotypes. Steeper slope of amplitude and frequency relation between sEPSCs and mEPSCs in GCs of A30P α-SYN mice indicates lower sensitivity of the sEPSCs amplitude to TTX. Values are presented as mean±s.e.m. Student’s t -test ( c , d ). Full size image This study presents converging evidence for detrimental effects of human A30P α-SYN on the development and synaptic integration of adult-born GCs in the mouse OB. It pinpoints the apical dendrites with dendro-dendritic synapses between developing GCs and resident MCs/TCs as the primary site for action of A30P α-SYN, which interferes with spine stability and dendrite growth and branching. While the latter render the developing GCs electrically more compact and hyper-responsive to depolarizing inputs, reduced stability and density of spines during the critical window of development hampers the engagement of new GCs into existing networks. Of note, the network-driven excitatory synaptic drive (sEPSCs) in adult-born GCs under the excess of noxious A30P α-SYN remains unaltered while mEPSCs display reduced frequency and enhanced amplitude. Thus, for the first time evidence is provided for specific developmental and functional impairments in adult-born GCs in A30P α-SYN mice, which may contribute towards their reduced survival [35] , [36] . On the functional side, the loss of GCs and changes in their intrinsic excitability and excitatory inputs shown here may disrupt the network dynamics in the OB and possibly contribute to the olfactory deficit—a well-recognized forerunner of the slower advancing motor impairments in the course of PD. Despite that the majority of PD mouse models fail to replicate the severe motor deficit resultant from the breakdown of the nigrostriatal dopaminergic system, they mimic the main traits of cellular pathology associated with harmful human α-SYN. One of the most common findings from these models is the reduced survival of adult-born neurons in the OB [35] , [36] , confirmed also by our data. There is growing evidence for a causative link between the level of PD-specific α-SYN in different brain regions and loss of residing therein nerve cells, with adult-born neurons in the OB and hippocampal dentate gyrus being especially vulnerable [5] . Noteworthy, however, neither functional alterations preceding the neuronal loss nor the underlying mechanisms have been identified. It emerges that the adult-born OB neurons are highly sensitive to disruptive effects of mutant α-SYN throughout their entire lifetime, from proliferation stage through maturation and integration into existing networks [5] , [35] , [36] . Considering the late expression of A30P α-SYN in our model, presumably owing to delayed onset/activation of the Thy1-promoter [23] , [24] , the effects of α-SYN shown herein are expected to be resultant of impaired integration of new GCs into α-SYN-loaded existing networks. Such interpretation accords with our recent findings of strong accumulation of phosphorylated A30P α-SYN in MCs [25] , and by the fact that the dendritic spine dynamics of new GCs strongly depend on MC feedback [31] , [32] . The presence of pathological A30P α-SYN in presynaptic terminals as well as in α-SYN-positive neuritic swelling in this model [23] implies that A30P α-SYN, like its normal variants, is trafficked to prime sites of its function—the synapse [37] , [38] . The latter, in addition to confirming the main functionality of this molecule as a key regulator of soluble NSF attachment protein receptor (SNARE)-driven membrane fusion, also implicates synaptic hotspots and ectopic fusion sites as principal targets of harmful α-SYN. Because the aggregates of oligomeric and fibrillar α-SYN can sequestrate the unfolded wild-type α-SYN [39] , exacerbation of the pathology with loss of GCs under the excessive A30P α-SYN in the OB is not surprising. Such possible loss-of-function effect is reflected in partial phenotypic convergence between A30P α-SYN and α-SYN KO genotypes. The milder synaptic effects of α-SYN deficiency with physiological survival of adult-born GCs in α-SYN KO mice, conceivably, can be explained by its substantial redundancy and functional overlap with other SYN (β- and γ-) variants [37] . This may also apply to the parameters of apical dendrites and spine dynamics in α-SYN KO, which, unlike A30P α-SYN, remained largely unchanged. On the other hand, the twofold prevalence of A30P α-SYN protein species in our model as compared with endogenous protein levels [23] is likely to have adverse effects on dendrite and spine dynamics, via other yet unknown mechanisms. Overall, it appears that a precise balance in α-SYN forms is imperative for maturation and integration of adult-born GCs into the existing circuits. While studies of human brain autopsy and animal models of PD have reported motor deficit associated with shrinkage of dendrites, 30–50% reduction in spine density and abnormal spine morphology in medium spiny neurons of the paleo- and neostriatum [40] , [41] , our data provide the first clear-cut evidence for related changes in adult-born GCs of OB. Given that the pathological process starts many years before the onset of motor symptoms, identification of the changes that underlie the early loss of bulbar neuron could foster better understanding of the pathobiology of the disease with its early diagnosis. Selective deposition of toxic α-SYN in the OB, but not in other forebrain structures, during pre-motor phase of PD [18] , [42] with extensive loss of new GCs renders this part of the brain an attractive experimental model [5] . Reduced dendrite outgrowth with spine deficit in GCs in A30P α-SYN mice reported in our work concur with the importance of α-SYN in promoting the regulated SNARE-driven membrane fusion [37] , [38] , [43] and structural plasticity. As the most dynamic and functionally demanding compartment of adult-born GCs, the apical dendrites require constant membrane expansion and turnover involving dendritic SNAREs [44] . Such a role of α-SYN, along with chaperoning the polymerization of microtubule-associated proteins and regulation of actin dynamics [45] would undoubtedly impair the spine stability, activity-dependent dendritic plasticity and dendrite growth [46] , [47] . It seems likely that during the critical phase of development and synapse formation in new GCs [31] , [32] , noxious α-SYN disrupts the fine processes warranting the adequate integration of new GCs into the existing OB networks, dooming them to death. This notion is consistent with related findings reported in adult-born GCs of the hippocampal dentate gyrus, where overexpression of wild-type α-SYN affects not only the complexity of dendritic arbours but also the density of mushroom spines [47] . In another model, also overexpressing abnormal α-SYN, the loss of adult-born GCs was preceded by deficiency of presynaptic markers [36] , [48] . Interestingly, sensory deprivation in rat pups was shown to cause substantial reduction in the dendritic expansion and spine density in OB adult-born GCs, leading to their hyper-excitability [49] . Such observations are in line with our earlier findings of impaired odour discrimination in A30P α-SYN mice [25] , and point to disruption of the MC–GC cross-talk as a major determinant for proper development of GC dendrites and spines. Conceivably, the unique characteristics of dendro-dendritic synapses with soaring membrane turnover at both GABA and glutamate release sites and high demand for structural plasticity render adult-born GCs especially vulnerability to the pathological α-SYN, affecting their functional integration and survival. From the perspective of synaptic integration and generating time-variant outputs by adult-born GCs, the decrease of electrical capacitance and increased resistance due to retarded dendrites are likely to alter their integrative properties. Indeed, reduced R in and C m of GCs due to underdeveloped dendrites can decrease the signal-to-noise ratio via conversion of the sub-threshold synaptic noise into a signal [50] . The latter, in turn, would promote indiscriminate inhibition and interrupt the output of MCs/TCs [51] . In the presence of TTX, the vast majority of events recorded in GCs are likely to be driven by spontaneous release of glutamate at dendro-dendritic contacts, with somatic inputs activated by recurrent collaterals [6] , [34] being suppressed, owing to their reliance on MC firing. While the reason for faster synaptic currents in our study compared with those reported earlier [35] remains unclear, both age and temperature-dependent acceleration of mEPSC kinetics [52] , [53] are likely to contribute. Of note, close to normal rate and amplitude of AMPA-receptor-mediated sEPSCs, together with the more potent effects of TTX in GCs of A30P α-SYN mice are consistent with increased activity of MCs/TCs and/or augmented responsiveness of excitatory inputs in new GCs of transgenic A30P α-SYN mice. Although the diminished length of dendrites with better space clamping [54] in GCs of A30P α-SYN mice might to some extent account for the larger amplitude of their mEPSCs, our data cannot rule out alterations of the expression and sensitivity of AMPA receptors [55] . Similar density of GluR1-positive clusters co-localizing on adult-born GC dendrites with a trend towards enlarged spine heads under reduced spine density point to this direction. It is worth mentioning that a small fraction of synapses can be immunonegative despite significant expression of receptors [56] , an experimental observation that would explain the observed discrepancy between glutamatergic and GABAergic inputs on new GCs. Our results thus highlight the essential role of dendro-dendritic integration for spine stability and survival. Together with impaired dendrite growth, these morphological and functional alterations caused by pathological α-SYN might lead to a reduced survival of adult-born GCs and hence olfactory disturbances. Animals, viral injections and open-skull craniotomy Young adult (2–6 months old, n =86) male wild-type (control), transgenic (A30P α-SYN expressed under the Thy1-promoter) [23] and α-SYN KO mice [57] of the same C57Bl6 background were housed (21±2 °C, humidity 36±2% at 12/12-h light/dark cycle; max. 5 mice per cage) and bred in the animal housing facility at the Center for Neuropathology and Prion Research, Ludwig Maximilian University Munich (LMU), with food and water provided ad libitum . All experimental procedures were approved by the local authorities and upper Government of Bavaria (Az. 55.2-1-54-2531-184-09). The presence of the transgenes of interest was verified using PCR with priers: (human A30P α-SYN : forward 5′-ATGGATGTATTCATGAAAGG-3′ and reverse 5′-TTAGGCTTCAGGTTCGTAG-3′; mouse α-SYN : forward 5′-CTGAATGAACTGCAGCAGCA-3′ and reverse 5′-ATACTTTCTCGGCAGGAGCA-3′). Replication-deficient LV encoding eGFP under control of the CAG promoter used for labelling adult-born neurons in the OB in vivo were produced [58] . In brief, HEK293 cells were transfected with the LV vector and helper plasmids (provided by Dr Michalakis, LMU) using the calcium phosphate transfection method. The primed medium was subsequently collected (48 and 72 h), the viral mass concentrated with ultracentrifugation and re-suspended in sterile Hank’s balanced salt solution. Intra-cerebral injections and open-skull craniotomy with implantation of chronic window over the OBs were carried out in mice deeply anesthetized with intraperitoneal (i.p.) injection of ketamine/xylazine (130 and 10 mg kg −1 body weight, respectively); dexamethasone (0.02 ml, 4 mg ml -1 ) was administered i.p. before the surgery. The stereotactic bilateral infusion of the LV (300–500 nl at a titre of ~10 8 infecting units per ml) into the RMS (A-3.3, L-0.8 and D 2.9 mm) were carried out according to the described protocol [27] , which was followed by craniotomy with implantation of a chronic window over both OBs, using established methods [59] . In brief, the skull was exposed and a 3-mm round hole was carefully opened with a dental drill. The exposed brain was cleaned with sterile saline and covered directly with a round cover-glass ( D =3 mm); the margin between the glass and skull was sealed with dental cement and glue (CyanoVeneer). A z-shaped holder was firmly attached to the skull for securing the head of the animal in the custom-made head holder. Post-surgical mice were subcutaneously injected with carprofen (Pfizer) and cefotaxime (Pharmore) (4 mg and 250 mg kg −1 , respectively) and allowed to fully recover before the start of the imaging (3–4 weeks post surgery). Mice (17/30) with windows of poor quality were not included in current analysis. Histology and confocal microscopy The survival of adult-born neurons in the OB was assessed through injections of BrdU (50 mg kg −1 , i.p.) over 5 consecutive days, with animals killed under deep anaesthesia at 21 or 32 days after the first BrdU injection [35] . Proliferation of neural precursors in the SVZ was estimated after injection of a single dose of BrdU (100 mg kg −1 , i.p. ), followed by brain removal after 24 h and quantification of labelled cells. Six-month-old mice received a lethal dose of ketamine (200 mg kg −1 ) and were perfused transcardially (phosphate-buffered saline (PBS), 50 ml), followed by 4% paraformaldehyde (150 ml). Brains were post-fixed in paraformaldehyde at 4 °C (8 h) with coronal sections of both OBs (50 μm) cut with microtome (VT 1000S, Leica). Freely floating sections were incubated in 5% normal goat serum, 1% bovine serum albumin and 0.1% Triton X-100 in PBS for 60 min at room temperature, followed by their exposure to primary antibodies at dilutions: mouse anti-NeuN (1:200) and rabbit anti-GluR1 (1:200) from Millipore, rat anti-BrdU (1:200) and rabbit anti-DCX (1:500) from Abcam, rabbit anti-VGAT (1:500) and mouse anti-Gephyrin (1:200) from Synaptic Systems, rabbit anti-GFP tagged with Alexa 488 (1:200) from Invitrogen. After several washes with PBS (0.1 M), all slices were incubated in corresponding secondary antibodies at dilution 1:500 for 4 h followed by their mounting with fluorescent mounting media and covered. Fluorescence images were acquired through the × 10 and × 40 NA oil immersion objectives in frames, using LSM 510 confocal microscope (Carl Zeiss). Laser lines used for excitation and range of collection of emitted signals were as follows: Alexa488/eGFP-488 nm/500–550 nm; Alexa647–633 nm/long-pass 650 nm and DAPI-750 nm/435–485 nm (two-photon excitation). Analysis of dendritic spines was limited to GC apical dendrites within the external plexiform layer, cropped and imaged at high resolution. For unambiguous analysis of LV GFP-labelled neurons, the slices were re-stained with anti-GFP antibody; same sections were used for morphometric analysis of dendritic expansion and branching. In vivo two-photon imaging In vivo two-photon imaging of adult-born GCs was performed in anaesthetized mice (ketamine 100 mg kg −1 and xylazine 7.5 mg kg −1 , i.p.) through open-skull cranial windows, using a LSM 7MP upright microscope (Carl Zeiss) equipped with a × 20/1.0 NA objective. The mouse was placed in a custom-made holder attached to the microscope stage with the head fixed and oriented consonantly relative to the objective, with an image of the blood vessel map acquired to ensure the return to the same imaging field in consecutive experiments. After imaging (45–60 min), the animal was returned back to its housing cage for rest. Data presented are from 5 consecutive imaging sessions from 17 mice, divided into 2 cohorts: the first underwent daily imaging from 21 up to 25 days post injection (d.p.i. ), on daily basis ( n =8; 51 dendrites); the second cohort was imaged from 28 up to 44 d.p.i. once every 4 days ( n =9; 39 dendrites). Neuronal eGFP was excited with a Mai Tai laser (DeepSee, Spectra-Physics) at 880 nm, with emitted photons collected and sampled through a photomultiplier detector module (NDD, LSM 7MP). Individual dendrites were imaged at 0.08 μm pixels resolution in xy and 1 μm in z dimensions. Efforts were made to keep the eGFP fluorescence constant throughout the entire experimental session. Image processing and data analysis For data analysis, only microscope image data with sufficient LV-eGFP expression and good signal-to-noise ratio were included. Dendritic trees of adult-born GCs were reconstructed from confocal image stacks to analyse the total dendritic length/branching and soma size using Neurolucida (MicrobrightField, USA). Counting of GABAergic synapse density was conducted on deconvoluted images (AutoQuantX2, Media Cybernetics). VGAT-, gephyrin- and GluR1-positive labelled elements (putative synaptic contacts) overlapping with eGFP-labelled dendrites were analysed with custom-written scripts (Igor Pro, Wavemetrics Inc., Lake Oswego, OR, USA) with threshold for distinguishing the fluorescence signal from noise set at 20% of the peak intensity of the signal [60] . The length of individual dendrites was measured manually with each spine identified along the dendrite tagged and scored as gained, lost or stable. The mean density of dendritic spines was estimated for each time point and expressed over 1 μm of dendrite length. The net change in spine density was quantified over time relative to the first imaging session. The stability of spines was calculated based on the amount of spines that remained unaltered for at least two subsequent imaging sessions. The spine turnover rate was assessed based on gain and loss of spines over each day of imaging, calculated as TOR=( N gained + N lost )/(2 × N present )/ I t , where N gained , N lost and N present represent the number of gained, lost or total spines at time points of interest, respectively, while I t is the number of days between consecutive imaging sessions. Morphological classification of dendritic spines was performed semi-automatically from maximal projection images of in vivo two-photon stacks, using Imaris 5.0.1 (Bitplane). All spines along the dendrite were marked and categorized into three different classes, according to established criteria [61] . Electrophysiological recordings Whole-cell recordings were made in acute OB slices from eGFP-labelled GCs from 6-month-old mice that received a single injection of eGFP LV into the RMS. Between 30 and 35 d.p.i., mice were anaesthetized with isoflurane and decapitated with the forebrain and OBs dissected out and placed for 5–6 min in ice-cold bubbled (95% O 2 , 5% CO 2 ) slicing solution (in mM): sucrose, 75; NaCl, 85; KCl, 2.5; NaH 2 PO 4 , 1.25; NaHCO 3 , 25; CaCl 2 , 0.5; MgCl 2 , 4; glucose, 25, pH 7.4. Subsequently, the tissue was glued to the adaptor fixed in the slicing chamber of the microtome (VT1200S; Leica) filled with the same solution. The OB slices were cut horizontally (250 μm) and transferred into a warming chamber (35 °C) for 30 min that was filled with the same solution except that sucrose was omitted and NaCl was increased to 125 mM. Afterwards, the slices were transferred into recording artificial cerebro-spinal fluid (in mM): NaCl, 125; KCl, 2.5; NaH 2 PO 4 , 1.25; NaHCO 3 , 25; CaCl 2 , 2; MgCl 2 , 2; glucose, 25 were being maintained at room temperature with continuous bubbling (95% O 2 , 5% CO 2 ). Recordings were made in the recording chamber fixed to the stage of an Olympus BX51 microscope under continuous perfusion, at 35±1 °C, with adult-born GCs visualized with differential interference contrast and epifluorescence optics using adequate Alexa488/GFP and Alexa574/Cy3 filters. Fluorescence images were obtained using a CCD camera (Photonix). Criteria for including GCs into the current analysis were (1) expression of eGFP, (2) generation of overshooting action potentials in response to depolarizing stimulus and (3) input resistance exceeding 300 MΩ. The analogue signals were filtered at 5 kHz (Bassel filter), digitally sampled at 10 kHz and stored for offline analysis (PatchMaster, EPC10USB). Patch pipettes were pulled from borosilicate glass (HEKA Electronics) using P87 puller (Sutter instruments) filled with a K-methyl sulfate-based internal solution containing (in mM): KCH 3 O 3 S, 140; KCl, 10; NaCl, 5; MgATP, 2; EGTA, 0.01; HEPES, 10; 280–290 mOsm, pH 7.3, with in-bath input resistance of 6–8 MΩ; Alexa594 (~0.5%; Invitrogen) was routinely supplemented to the internal solution. Membrane potential was corrected for liquid junction potential of +8 mV. The input resistance and membrane capacitance ( R in and C m , respectively) were assessed using hyperpolarizing voltage steps of −5 mV, from a holding potential of −65 mV. Series of depolarizing pulses of 1,000 ms (5 mV increments) were used to induce action potentials. Synaptic currents were analysed offline with Mini Analysis (Synaptosoft, GE); current traces were smoothed ( × 5 binomial filter); the threshold defining synaptic events was set 2.5–3 times the s.d. of the baseline noise. Events were detected automatically and were occasionally re-examined by eye to exclude false-positive results. Curves were fitted and graphs were generated in IgorPro (WaveMetrics Inc.). Broad spectrum ionotropic glutamate (kynurenic acid, 5 mM), NMDA (D-AP5, 50 μM) and GABA A receptor (picrotoxin 200 μM) blockers were used to inhibit the synaptic activity. The mEPSCs were isolated by blockade of action potential-dependent synapse activity with TTX (0.5 μM, Biotrend). Statistical analysis and data presentation All data were analysed in a blinded manner using randomly assigned codes for control and experimental groups. Sample size was assessed based on the power of a hypothesis test. Two-way analysis of variance followed by the Bonferroni post hoc test was used to compare the variance of spine parameters assessed over time points of interest in two groups (control and A30P α-SYN). Changes within one group over time were statistically evaluated with one-way analysis of variance followed by the Tukey–Kramer post hoc test. Multiple comparisons between genotypes were also performed with the same test. The distribution of spine morphology classes was statistically rated using the χ 2 -test. In the rest of experimental data, Student’s t -test (unpaired, two-sided) was applied for assessment of inter-group differences at single time points and electrophysiological readouts from different genotypes. All structural data were tested for normal distribution. Data are expressed as mean±s.e.m. unless otherwise indicated, with P <0.05 defining differences as statistically significant (* P <0.05; ** P <0.01; NS=not significant). How to cite this article: Neuner J. et al. Pathological α-synuclein impairs adult-born granule cell development and functional integration in the olfactory bulb. Nat. Commun. 5:3915 doi: 10.1038/ncomms4915 (2014).